Global warming favours light-coloured insects in Europe Associations between biological traits of animals and climate are well documented by physiological and local-scale studies. However, whether an ecophysiological phenomenon can affect large-scale biogeographical patterns of insects is largely unknown. Insects absorb energy from the sun to become mobile, and their colouration varies depending on the prevailing climate where they live. Here we show, using data of 473 European butterfly and dragonfly species, that dark-coloured insect species are favoured in cooler climates and light-coloured species in warmer climates. By comparing distribution maps of dragonflies from 1988 and 2006, we provide support for a mechanistic link between climate, functional traits and species that affects geographical distributions even at continental scales. Our results constitute a foundation for better forecasting the effect of climate change on many insect groups. During the last decades, considerable interest has arisen in predicting the distribution of species, assemblages of species and characteristics of assemblages under various scenarios of climate change [1] , [2] , [3] , [4] . Most of these predictions, however, are based on phenomenological models [5] and provide little mechanistic understanding of the underlying processes [6] . A first step towards understanding the impact of climate change is to consider traits of species that underpin the relationship between species and climate [7] . This approach has been very successful for plants. For instance, leaf size as well as leaf shape have been used to reconstruct temperature and precipitation of paleoclimates [8] . However, the relationships between traits of animals and climate are more difficult to identify. One trait—the body size of endotherms—may be related to climate. Bergmann’s rule predicts a decrease in their body size within species and across closely related species with increasing temperature [9] , [10] . In line with this ecogeographic rule, a recent study found that the body size of some mammals decreases with increasing temperature [11] . Although many physiological and local-scale studies on insects have demonstrated associations between traits and climate, to what extent such mechanistic links may impact distribution patterns of insect species at a biogeographical scale remains largely unknown (but see ref. 12 ). In ectotherms, the appearance of the body surface and in particular its colour value are involved in thermoregulation [13] . Dark-coloured ectotherms are able to increase their body temperatures above ambient air temperature more effectively than light-coloured ectotherms, and therefore have an advantage in cool climates (thermal melanism hypothesis [14] , [15] ). Most insects—by far the most species-rich lineage of ectotherms [16] —need to reach body temperatures above ambient temperature for flying, foraging or mating [17] . However, being dark is only advantageous in cool climates. In areas with high temperatures and insolation, insects need to protect themselves against overheating [18] . At high temperatures, ectothermic species with light colouration can be active for a longer period than species with dark colouration, and may be able to use a broader thermal range of habitats. Overall, heat avoidance and heat gain constraints lead to the prediction that insect assemblages should be dominated by dark-coloured species in cool climates and by light-coloured species in warm climates. The first hint that this holds even at a biogeographical scale was provided by Rapoport [19] almost 50 years ago, when he used a rough estimate of springtail colour value to show a positive correlation of the percentage of dark-coloured species in species assemblages with latitude and altitude. In this study, we combine recent digital image analysis and phylogenetic statistics to demonstrate that colour lightness of insects is consistently correlated to the thermal environment across Europe. We furthermore show that assemblages of dragonflies became on average lighter-coloured during the last century, which we attribute to global warming. Mechanistic adaptation of species to climate Using a data set of nearly all European butterfly and dragonfly species, we show that insect species with dark and light colouration have advantages in cool and warm climates, and that this mechanistic adaptation of species to climate shapes the biogeographical patterns of species distributions. The results were obtained by measuring the colour value of the body and the dorsal and ventral basal wing areas of 366 butterfly species occurring in Europe using computer-assisted digital image analysis and the colour value (further on called colour lightness) of the body of 107 dragonfly species of Europe. The dorsal surface of butterflies was on average darker than the ventral surface, and the colour lightness strongly differed between families in both groups ( Supplementary Figs 1 and 2 ; and Supplementary Tables 1 and 2 ). All statistical approaches consistently showed that the mean colour lightness of assemblages increased with a synthetic variable that characterized the thermal environment within grids, that is, colour lightness increased with increasing temperature ( Fig. 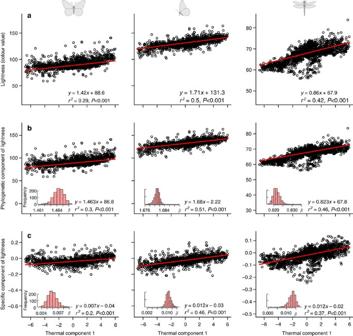Figure 1: Scatterplots of the different measures of the average colour value of butterfly and dragonfly assemblages versus our thermal component 1. This component is a variable that summarizes the thermal environment within each grid from cool (low values) to warm (high values). Note that for all measures of colour value as well as for the two groups of insects, the colour lightness of assemblages is consistently correlated to the thermal environment. (a) Average colour values across species on a scale from 0 (black) to 255 (white). (b) Average phylogenetic component, that is, the predicted colour value of each species based on the phylogeny. (c) Average specific component, that is, the deviation from the colour value expected by the phylogeny. Parameters are from univariate regression models weighted with the number of species in each grid cell (butterflies:n=1,825; dragonflies:n=1,845). The inserted histograms are represented as lines inbandcshow the distribution of regression slopes (β) calculated for 1,000 alternative phylogenetic trees. These regressions were all highly significant (t-test,P<0.001) with positive slopes throughout, indicating that the positive relationship between colour lightness and the thermal environment is robust to uncertainties in the phylogenetic trees. 1 , Table 1 ). These results support a mechanistic link between climate and functional traits of species, and indicate that an ecophysiological phenomenon can cause noticeable biogeographical patterns of insects ( Fig. 2 ). Figure 1: Scatterplots of the different measures of the average colour value of butterfly and dragonfly assemblages versus our thermal component 1. This component is a variable that summarizes the thermal environment within each grid from cool (low values) to warm (high values). Note that for all measures of colour value as well as for the two groups of insects, the colour lightness of assemblages is consistently correlated to the thermal environment. ( a ) Average colour values across species on a scale from 0 (black) to 255 (white). ( b ) Average phylogenetic component, that is, the predicted colour value of each species based on the phylogeny. ( c ) Average specific component, that is, the deviation from the colour value expected by the phylogeny. Parameters are from univariate regression models weighted with the number of species in each grid cell (butterflies: n =1,825; dragonflies: n =1,845). The inserted histograms are represented as lines in b and c show the distribution of regression slopes ( β ) calculated for 1,000 alternative phylogenetic trees. These regressions were all highly significant ( t -test, P <0.001) with positive slopes throughout, indicating that the positive relationship between colour lightness and the thermal environment is robust to uncertainties in the phylogenetic trees. Full size image Table 1 Multiple regression models between characteristics of the climate within grid cells and mean phylogenetic and specific components of butterfly and dragonfly colour lightness in Europe. 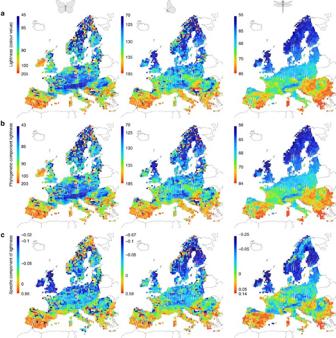Figure 2: Average colour value of butterfly and dragonfly species in Europe. (a) Average colour values across species on a scale from 0 (black) to 255 (white). (b) Average phylogenetic component, that is, the predicted colour value of each species based on the phylogeny. (c) Average specific component, that is, the deviation from the colour value expected by the phylogeny. The colour code of the individual maps is adjusted according to the specific values of each grid following equal-frequency classification; red indicates light-coloured assemblages and blue indicates dark-coloured assemblages (butterflies:n=1,825; dragonflies:n=1,845). For the raw colour value, the phylogenetic as well as the specific component, we found a decrease from assemblages dominated by light-coloured species in the south to assemblages dominated by dark-coloured species in the north. Full size table Figure 2: Average colour value of butterfly and dragonfly species in Europe. ( a ) Average colour values across species on a scale from 0 (black) to 255 (white). ( b ) Average phylogenetic component, that is, the predicted colour value of each species based on the phylogeny. ( c ) Average specific component, that is, the deviation from the colour value expected by the phylogeny. The colour code of the individual maps is adjusted according to the specific values of each grid following equal-frequency classification; red indicates light-coloured assemblages and blue indicates dark-coloured assemblages (butterflies: n =1,825; dragonflies: n =1,845). For the raw colour value, the phylogenetic as well as the specific component, we found a decrease from assemblages dominated by light-coloured species in the south to assemblages dominated by dark-coloured species in the north. Full size image Phylogenetic and specific components of colour lightness The colour lightness of each species has two components: a phylogenetic component and a species-specific component. The phylogenetic component is in part determined by the response of the ancestors to paleoclimates, whereas the species-specific response measures the deviation of each species from the ancestors. The latter component is therefore the more recent response of species to environmental factors. When we considered these two components, we found a clear decrease in the mean colour lightness of insect assemblages for both the mean phylogenetic components and the species-specific components across Europe from the Mediterranean to Northern areas. This result was consistent for the ventral and dorsal surfaces of butterflies and for the dorsal surface of dragonflies (Figs 1 and 2 [1] , [2] , and Table 1 ). Impact of climate change on insects If colour lightness of assemblages across Europe is a reaction to climate, we would thus expect that climate change would lead to changes in the colour lightness of insect assemblages. To test this hypothesis, we compared recent distributional data of dragonflies with data before 1988 and plotted the shift of colour lightness within grids ( Fig. 3 ). After correcting for phylogeny, we found a general shift towards lighter-coloured assemblages across Europe ( Fig. 3c ). In the phylogenetic component ( Fig. 3b ), we found shifts towards darker assemblages along the western margin of Europe, the Alps and the Balkans. However, the variation in the phylogenetic component still contains a portion of ‘phylogenetically structured environmental variation’ [20] . In addition, the change in colour lightness was positively correlated to the change in annual mean temperature (AMT) between the time periods corresponding to the distribution data ( Fig. 4 ). However, we would like to stress that the strength of the shift depends on the models used. Alterations in the distributions of species result in a complex spatial pattern in the colour lightness of assemblages, which is a clear indication that the response of assemblages of organisms to climate change does not lead to simple one-dimensional shifts (see for example, the Alps and the Scandinavian Mountains). 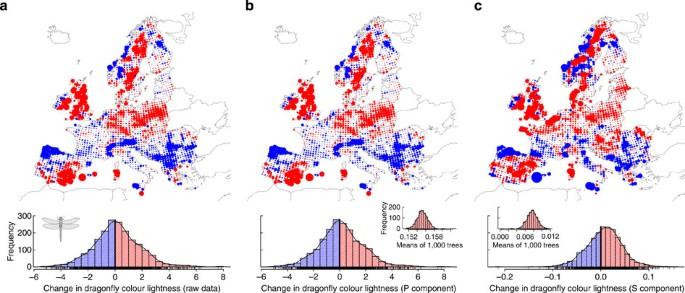Figure 3: Shift in the mean colour value of dragonfly assemblages across Europe between 1988 and 2006. Shift in colour value for (a) the raw data; (b) the phylogenetic component (P); and (c) the specific component (S). Red indicates an increase in colour lightness; blue indicates a decrease in colour lightness. The diameter of each dot indicates the extent of the shift (n=1,845). The distribution of the shifts shows for the specific component a clear trend towards higher (that is, lighter-coloured) values (peak of the distribution positive; zero indicated by black line). The phylogenetic component suggests that the shifts in colour lightness have a strong phylogenetic background leading to a complex geographic mosaic in the response of assemblages to climate change. The inserted histograms show the mean change in colour lightness calculated for 1,000 alternative phylogenetic trees and are positive throughout, indicating that uncertainties in the phylogenetic hypotheses are unlikely to affect our conclusion of a general shift towards lighter assemblages. The distributional information used in the analysis is often based on a large time span, that is, the distributional information published in 1988 summarizes data until that year using information even from the beginning of the twentieth century. Rugs at the abscissa indicate observed values. Figure 3: Shift in the mean colour value of dragonfly assemblages across Europe between 1988 and 2006. Shift in colour value for ( a ) the raw data; ( b ) the phylogenetic component (P); and ( c ) the specific component (S). Red indicates an increase in colour lightness; blue indicates a decrease in colour lightness. The diameter of each dot indicates the extent of the shift ( n =1,845). The distribution of the shifts shows for the specific component a clear trend towards higher (that is, lighter-coloured) values (peak of the distribution positive; zero indicated by black line). The phylogenetic component suggests that the shifts in colour lightness have a strong phylogenetic background leading to a complex geographic mosaic in the response of assemblages to climate change. The inserted histograms show the mean change in colour lightness calculated for 1,000 alternative phylogenetic trees and are positive throughout, indicating that uncertainties in the phylogenetic hypotheses are unlikely to affect our conclusion of a general shift towards lighter assemblages. The distributional information used in the analysis is often based on a large time span, that is, the distributional information published in 1988 summarizes data until that year using information even from the beginning of the twentieth century. Rugs at the abscissa indicate observed values. 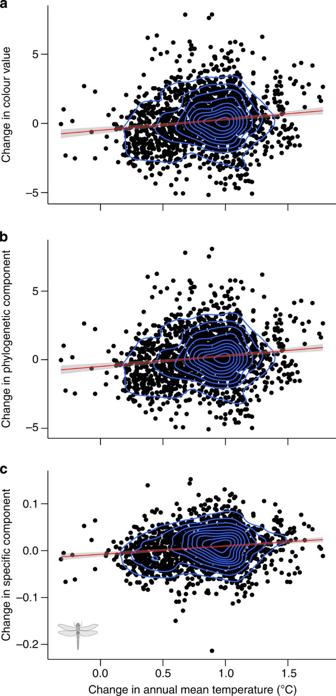Figure 4: Scatterplots of the shift in colour value of European dragonfly assemblages versus the change in annual mean temperature between the periods 1900–1988 and 1988–2006. Scatterplots are presented for (a) the raw data; (b) the phylogenetic component; and (c) the specific component. Each dot represents a 50 km × 50 km grid cell across Europe with density estimation (blue contours,n=1,845). Red lines are from ordinary regressions with 95% confidence intervals (grey shade). These regressions were all highly significant (t-test,P<0.001, see also Methods section) with positive slopes throughout, that is, dragonfly assemblages became lighter coloured in regions where temperature increased during the last century. Full size image Figure 4: Scatterplots of the shift in colour value of European dragonfly assemblages versus the change in annual mean temperature between the periods 1900–1988 and 1988–2006. Scatterplots are presented for ( a ) the raw data; ( b ) the phylogenetic component; and ( c ) the specific component. Each dot represents a 50 km × 50 km grid cell across Europe with density estimation (blue contours, n =1,845). Red lines are from ordinary regressions with 95% confidence intervals (grey shade). These regressions were all highly significant ( t -test, P <0.001, see also Methods section) with positive slopes throughout, that is, dragonfly assemblages became lighter coloured in regions where temperature increased during the last century. Full size image The interpretation of our results is conditional upon the assumption that thermoregulation is the predominant selective pressure for the evolution of wing or body colouration. However, colour lightness and colouration in general may be influenced by numerous other selective forces, for example, cryptic colouration [21] or disease and parasite resistance [22] . Our statistical models of butterflies showed that the positive relationship between the thermal environment and colour lightness is stronger for the ventral surface than for the dorsal surface ( Table 1 ), which suggests that selective pressures other than thermoregulation are more important for the colouration of the dorsal surface than of the ventral surface. A stronger relationship between colour lightness and ventral wing surfaces is not entirely surprising, since several species exclusively use the ventral surfaces for thermoregulation (for example, Colias and Gonepteryx ). Furthermore, ventral wing surfaces are additionally used for heat avoidance by reflecting insolation when wings are closed [23] . Despite these other potential pressures, the strong and consistent relationships between colour lightness and thermal environment across two insect groups underline the overall importance of climate for insects. After the last glaciation, butterflies and dragonflies recolonized wide areas of Europe, but most of the butterfly and dragonfly clades evolved before the Pleistocene [16] . The latitudinal gradient of the phylogenetic component suggests that exaptations [24] have been of considerable importance during the assembly of northern insect faunas after the last glaciation, that is, colour lightness might have evolved for or as a by-product of other functions in a different spatio-temporal selective regime. But the trends in the species-specific component indicate that the comparatively dark-coloured species of all clades colonized northern areas. Our finding that the assembly of insect faunas in response to the thermal environment depends on the colour lightness of certain body parts clearly demonstrates the importance of thermal energy in structuring insect assemblages—even across larger spatial scales. This has implications in forecasting the effect of climate change [1] , [2] , [3] , [4] , [5] , [6] , [25] , [26] , [27] . With global warming, we would thus expect that dark-coloured insects will shift their distribution and possibly retreat from certain areas [28] and/or on a smaller scale will shift their habitat preference to more shady conditions [29] . The latter scenario has consequences for conservation strategies : conservation efforts directed exclusively toward current habitat preferences without taking into consideration the effect of ecophysiological adaptation may be futile for the future as the climate changes. Distribution data We used distribution maps of 434 European butterfly species [30] . After matching these with the species illustrated in ref. 31 , we were able to consider 366 species across 1,825 grid cells of 50 km × 50 km. We created a database of 107 dragonfly species across 1,845 grid cells [32] ( Supplementary Tables 1–3 , and Supplementary Methods ). The butterfly distribution maps were presence/absence maps; the dragonfly distribution maps were outline maps. Computer-assisted digital image analysis Computer programs for the analysis of digital images provide possibilities to measure the colour value from scanned published illustrations [33] , [34] . We scanned ventral and dorsal butterfly wings and dragonfly bodies and converted the scanned RGB (red, green, blue) colour illustrations into 8-bit grey values. We assigned each pixel a value between 0 (complete black) and 255 (complete white), and averaged these values across all pixels of the considered area to obtain a single colour value for each species. Usually, software such as PhotoShop weights the three RGB channels according to the perception of human eyes when converting to grey values (for example, 0.21 × R+0.72 × G+0.07 × B). This is because some colours are subjectively perceived darker than others. For example, blue looks darker than green for humans at the same value of colour lightness. We decided to calculate the unweighted mean across the three RGB channels. Note that dark-coloured species have a low value and light-coloured species have a high value. In particular, we scanned the ventral and dorsal part of the wings of female butterflies illustrated in ref. 31 with an EPSON Perfection 4490 Photo Scanner with 1,200 dpi and 24 bit in the RGB colour spectrum. All further steps to estimate the colour value were done with Adobe Photoshop CS2, Adobe Photoshop Elements 2, Epson Scan Ver. 2.75G and ImageMagick 6.5.5-2. In our study, we predominantly considered females because their parental investment is higher and colouration of males may be biased by sexual selection [35] . Therefore, females can be expected to be closer to a ‘thermal optimum’. Only if an illustration of a female was not available, we used an illustration of the male (butterflies: 28 male and 338 female). Note that dorsal and ventral colour lightness was closely and significantly correlated between the sexes ( t -test, P <0.001 dorsal, ventral ; adjusted r 2 =0.62 dorsal , 0.9 ventral ; n =387 dorsal , 391 ventral , all available images). For butterflies, the most relevant part of the wing for thermoregulation is the wing area near the body [36] . Therefore, we decided to measure the body and 1/3 of the wing area closest to the body. We scanned the thorax and abdomen of dragonflies illustrated in ref. 37 . For some species, illustrations of both sexes were not available (74 of 114). To make use of as many species as possible, we solely processed dorsal drawings of male dragonflies. In doing so, we were able to use 107 of 114 dragonfly species presented in ref. 37 . Note that in ref. 37 , female drawings are often depicted from lateral, making comparisons difficult. Note also that beside these limitations, colour lightness of male and female species was significantly correlated ( t -test, P <0.001, adjusted r 2 =0.23, n =40 because of the limited availability of female drawings). For some species, the thorax was not drawn because they differ from each other only in shape and colour of the abdomen. In such cases, we composed the images of the abdomen with corresponding drawings ( Lestes viridis with the female image; Cordulegaster heros , C. picta and C. principes with C. boltoni ). All further calculations followed the procedure for butterflies. The colour value used in our study was derived from a three-channel evaluation of wing patterns in the visible spectrum and is therefore only a proxy for the overall properties. However, a major advantage of our method is the acquisition of standardized and hence comparable colour values. But it only gives information on pigment colouration, not structural colouration or iridescence (angel-dependent colour; for example, wings of some male Lycaenids), and values represent mean phenotypes without intra-specific variation. We tested the robustness of our procedure to estimate the colour value, and confirmed that the extracted values represent the physical ability of the species to absorb and reflect radiation energy ( Supplementary Methods ; and Supplementary Figs 3–5 ). Phylogenetic analysis We constructed phylogenies for butterflies and dragonflies ( Supplementary Methods ). Lynch’s comparative method [38] was used to partition the colour value of each species into a phylogenetic and a specific component. The phylogenetic component describes the part inherited from the ancestor; the specific component measures the deviation from the relatives. We decided to apply Lynch’s comparative method because it not simply ‘corrects’ for phylogeny but also partitions the trait phenotype into a phylogenetic and a non-phylogenetic part that can be used for further analyses. Furthermore, it has the advantage to allow to incorporate the phylogenetic signal [39] and different modes of evolution [40] in its correlation structure (for details, see refs 38 , 41 , 42 ). Lynch’s model describes the observed trait phenotype ( y i for the i th taxon) as the sum of a grand phylogenetic mean ( μ ), a heritable component ( a i ) and a residual deviation ( e i ): y i = μ + a i + e i . The grand phylogenetic mean μ is a scaling term that can be interpreted as the state of the ancestor at the root of the phylogeny. The quantity μ + a i is the predicted value by the phylogeny and can be interpreted as the phylogenetically heritable component of the observed phenotype of the i th taxon. It is termed ‘phylogenetic component’ in this article. Hence, the residual deviation e i from the phylogenetic component is termed ‘specific component’. Subsequently, we calculated for each grid cell in Europe the mean values of the phylogenetic and specific components of the subset of the occurring species. In addition, we used phylogenetic eigenvector regression [43] to disentangle the phylogenetic and the specific components of colour lightness and found similar results (not shown). Using Lynch’s comparative method, we addressed three fundamental evolutionary assumptions of phylogenetic approaches, namely that the phylogeny is constructed without error (phylogenetic uncertainty), that more closely related species tend to show more similar characteristics than expected by chance (phylogenetic signal), and that the evolutionary model used is appropriate (evolutionary model uncertainty) [44] . Phylogenetic uncertainty We resolved the multifurcations in our trees within a Bayesian framework using R and BEAST [45] as described in ref. 46 (see also refs 47 , 48 , 49 , 50 for recent developments in the field). We calculated two maximum clade credibility trees with mean node heights for butterflies and dragonflies and used these trees in subsequent phylogenetic analyses. To give more probabilistic support to our results, we randomly draw 1,000 trees from the BEAST output, repeated the analyses and checked for the robustness of the results (see inserted histograms in Figs 1 and 3 ). In particular, we calculated the phylogenetic signal lambda [51] , [52] and used this value to scale the phylogenetic correlation matrix (see refs 39 , 53 , 54 for examples within a phylogenetic generalized least-squares framework) in Lynch’s comparative method for each tree (see ref. 38 and functions corPagel and compar.lynch in the R package ape [55] ). Here, the correlation structure followed a Brownian motion model with the off-diagonal elements multiplied by lambda. Phylogenetic signal We calculated the phylogenetic signal (lambda) for every tree with fitContinuous in the R package geiger [56] version 1.99–3 and found high values of lambda, with higher values for butterflies than for dragonflies (median and mean >0.80; Supplementary Fig. 6 ). This indicates that related species have more similar colour lightness than expected by chance, and hence the phylogenetic variance–covariance matrix needs to be scaled by lambda [39] . When compared with the phylogenetic signal in body size—which we assume to be a key niche trait—there was even no significant difference to the ventral colour lightness of butterflies. However, potential micro-evolutionary causes of this pattern, for example, gene flow, pleiotropy or lack of genetic variability cannot be distinguished within the framework of this study. Evolutionary model uncertainty The resulting correlations of the trait values of species in the phylogeny can be seen as a function of an evolutionary model-specific transformation of the branch lengths of the original phylogeny. Following ref. 44 , a fundamental assumption of phylogenetic analyses is that the model of character evolution effectively recapitulates their history, and this implies to compare several evolutionary models. Hence, to support our main conclusions that (i) colour lightness is consistently correlated to the thermal environment, and that (ii) dragonfly assemblages became on average lighter-coloured during the last century, we simultaneously accounted for evolutionary model and phylogenetic uncertainty. However, we would like to highlight that it is not our intention to make statements about the most adequate model for the evolution of colour lightness in butterflies and dragonflies, so we arbitrarily chose four evolutionary models to underline the robustness of our conclusions: (i) the model ‘lambda’ [51] , [52] fits the extent to which the phylogeny predicts covariance among trait values for species by multiplying the off-diagonal elements in the correlation structure by the value of lambda. Interpreted as a tree transformation, values of lambda near 0 cause the phylogeny to become more star-like, and a lambda value of 1 recovers the Brownian motion model. Bounds for the estimation of lambda were set to 0 and 1. This model was used for the results presented in the main text. (ii) In the model ‘kappa’ [51] , character divergence is related to the number of speciation events between two species. Interpreted as a tree transformation, the model raises all branch lengths to the power kappa. Bounds for the estimation of kappa were set to 0 and 1. (iii) The Early-burst [57] or also called accelerating-decelerating (ACDC) [58] model is a model where the rate of evolution increases or decreases exponentially through time. Bounds for the estimation of the scaling parameter a were set to −10 and 10. (iv) The Ornstein–Uhlenbeck model [59] fits a random walk with a central tendency and an attraction strength proportional to the parameter alpha. Bounds for the estimation of alpha were set to 0 and 10 5 . Model parameters were estimated for 1,000 randomly selected phylogenetic trees in each model with the function fitContinuous in the R package geiger [56] version 1.99–3. All trees were transformed with their estimated parameters (function transform.phylo) and used to partition colour lightness into a phylogenetic and a specific component with Lynch’s comparative method [38] . For each tree, we calculated for each grid cell in Europe the mean values of the phylogenetic and specific components of the subset of the occurring species and regressed these values against our thermal component 1. Regarding our main conclusion (i) that colour lightness is consistently correlated to the thermal environment, we found that all 24,000 regressions were highly significant ( t -test, P <0.001) with positive slopes throughout the models, indicating that different evolutionary models do not alter the positive relationship between colour lightness and the thermal environment ( Supplementary Fig. 7 ). To give more probabilistic support to our main conclusion (ii) that dragonfly assemblages became on average lighter-coloured during the last century, we followed the procedure described above and calculated for each grid cell in Europe the mean value of the phylogenetic and specific components according to the dragonfly distributional information of 1988 and 2006. We calculated the change in colour lightness for each grid cell and averaged these changes across Europe for each tree and evolutionary model. We found the majority of values to be positive, indicating that different evolutionary models do not alter the overall shift towards lighter-coloured dragonfly assemblages ( Supplementary Fig. 8 ). Environmental variables For each grid cell across Europe, 25 environmental variables were extracted from public resources using Grass GIS version 6.4.0RC6. Since data were not available for all grid cells, the data set was reduced to grid cells for which information was available for all environmental variables (1,825 for butterflies and 1,845 for dragonflies). (i) Yearly sum of solar irradiation on horizontal surface (INS): in the data source used (ref. 60 , http://re.jrc.ec.europa.eu/pvgis/download/download.htm ), atmospheric corrections were already applied to account for spatial differences in, for example, average cloud cover, atmospheric turbidity and shadowing by the local terrain. (ii) Temperature-related variables: we used AMT, mean diurnal temperature range, isothermality, temperature seasonality, maximum temperature of warmest month, minimum temperature of coldest month, temperature annual range, mean temperature of wettest quarter, mean temperature of driest quarter, mean temperature of warmest quarter and mean temperature of coldest quarter to characterize the thermal environment. Data were taken from BioClim [61] , available at http://www.worldclim.org/current . (iii) Precipitation-related variables: since actual evapotranspiration is reported to be a strong predictor of species richness of European butterflies [62] , we considered annual precipitation, precipitation of wettest month, precipitation of driest month, precipitation seasonality, precipitation of wettest quarter, precipitation of driest quarter, precipitation of warmest quarter and precipitation of coldest quarter. Data were taken from BioClim [61] , available at http://www.worldclim.org/current . (iv) Topography-related variables: since precipitation and ambient temperature are related to topography, we used five measures describing the topography within each grid during subsequent analyses: average elevation, lowest elevation, highest elevation, elevation range and s.d. of elevation. Data are available at http://www.biochange-lab.eu/files/europe50km.zip [63] . Statistical analysis Our primary interest was to identify the strongest predictors of the mean colour value of butterfly or dragonfly species co-occurring within grids across Europe. Therefore, we applied a principal component analysis (PCA) based on the correlation matrix to reduce the dimensionality in the environmental variables [64] . We applied separate PCAs for the categories thermal environment, precipitation and topography. Of course this leads to correlated components across the separate PCAs. The idea was, however, to characterize the different aspects of the climate and naturally the different aspects are correlated (for example, topography and thermal environment). The PCAs extracted two components with eigenvalues >1 from the categories temperature and insolation, which characterize the thermal environment of the respective grid cell (Thermal 1 and 2), as well as two components for precipitation (Prec 1 and Prec 2) ( Supplementary Table 5 ). The PCA extracted one eigenvector (Topo) for the topography ( Supplementary Table 5 ). For temperature and precipitation, the first axis (called Thermal 1 and Prec 1) characterized the overall mean, and the second axis (Thermal 2 and Prec 2) characterized the variability of temperature or precipitation across the year. Since the directions of ecological associations between response and predictors in models with PCs are difficult to interpret because the sign of axis scores is arbitrary, we plotted selected variables of each category for illustration ( Supplementary Fig. 9 ). We calculated multiple regression models using the phylogenetic and specific components of the mean colour value within grids and the principal components of the environmental variables. Assumptions of an ordinary least-squares regression are that the standard error of the error term is constant over all values of the response, and that explanatory variables and all estimates provide equally precise information. Because the standard error of the calculated mean colour value of assemblages within grids differed in relation to the number of species recorded within grids, using the number of species per grid cell as weights to the least-squares regression improves parameter estimation (see also ref. 65 ). To further improve the information quality of the data, we included only grid cells in the analysis of butterflies with more than five recorded species. To account for spatial autocorrelation in the model residuals after fitting the environmental components to the data, we build spatial simultaneous autoregressive models, where the error term is predefined from a spatial neighbourhood matrix, and autocorrelation in the dependent variable is modelled within a generalized least-squares framework using maximum likelihood [66] . Calculations were performed with the function errorsarlm in the R package spdep version 0.5–65 for neighbours within 1,000 km distance. We applied hierarchical partitioning to assess whether multicollinearity between the PCs of the different categories might affect the results. Hierarchical partitioning decomposes the variation contained in a response variable into independent parts, which reveal the absolute importance of each predictor by considering all possible variable combinations in a hierarchical multivariate regression setting [67] . Calculations were performed in R with the package hier.part version 1.0–3 using ‘ r 2 ’ as the goodness-of-fit measure. We also included phylogenetic and specific parts of body size (digitally measured fore-wing length of butterflies and body length of dragonflies) in the analysis. We found qualitatively similar results compared with the findings of Table 1 , indicating that multicollinearity and body size does not change our main results ( Supplementary Fig. 10 ). All statistical analyses were performed with the software R ( www.r-project.org ). Intensive calculations were conducted using the MaRC2 High Performance Computing cluster in Marburg. Change in dragonfly colour lightness To analyse changes in the colour value of dragonfly assemblages, we compared the data used in our statistical analysis (distribution of 2006, ref. 32 ) to maps of the distributions before 1988 (ref. 37 ), and plotted the distribution of the shift in colour lightness within grids and the average shift across all grids for multiple phylogenetic trees ( Fig. 3 ). In addition, we extracted climatic data corresponding to the two distribution data sets of dragonflies in Europe from public resources (CRU TS3.2, ref. 68 ). We calculated the AMT for the period 1900–1988 and for 1988–2006; determined the change in AMT between these two periods; and correlated this change to the change in colour lightness of dragonfly assemblages ( Fig. 4 ). We found positive correlations ( t -test, P <0.001) for the raw data, the phylogenetic component and the specific component of colour lightness. Correlations using simultaneous autoregressive models to incorporate spatial autocorrelation were also all significant ( t -test, P <0.05) and positive. This indicates that dragonfly assemblages became lighter coloured in regions where temperature increased during the last century, giving further support to our conclusion that climate warming favours light-coloured insects in Europe. How to cite this article: Zeuss, D. et al. Global warming favours light-coloured insects in Europe. Nat. Commun. 5:3874 doi: 10.1038/ncomms4874 (2014).